The E3 ubiquitin ligase Trim7 mediates c-Jun/AP-1 activation by Ras signalling The c-Jun/AP-1 transcription factor controls key cellular behaviours, including proliferation and apoptosis, in response to JNK and Ras/MAPK signalling. While the JNK pathway has been well characterized, the mechanism of activation by Ras was elusive. Here we identify the uncharacterized ubiquitin ligase Trim7 as a critical component of AP-1 activation via Ras. We found that MSK1 directly phosphorylates Trim7 in response to direct activation by the Ras–Raf–MEK–ERK pathway, and this modification stimulates Trim7 E3 ubiquitin ligase activity. Trim7 mediates Lys63-linked ubiquitination of the AP-1 co-activator RACO-1, leading to RACO-1 protein stabilization. Consequently, Trim7 depletion reduces RACO-1 levels and AP-1-dependent gene expression. Moreover, transgenic overexpression of Trim7 increases lung tumour burden in a Ras-driven cancer model, and knockdown of Trim7 in established xenografts reduces tumour growth. Thus, phosphorylation–ubiquitination crosstalk between MSK1, Trim7 and RACO-1 completes the long sought-after mechanism linking growth factor signalling and AP-1 activation. The Ras signalling pathway regulates a large and diverse array of cellular decisions, including cell proliferation. Around 30% of all human tumours harbour activating mutations in Ras or its downstream kinases, which contribute towards several aspects of the malignant phenotype such as deregulated growth, apoptosis and invasiveness [1] , [2] , [3] . Oncogenic Ras induces constitutive activation of many effectors that are normally activated by growth factor stimulation, driving cell growth and proliferation [1] . Among these effects is the upregulation of c-Jun, a member of the AP-1 transcriptional activator family, which controls transcription of cell cycle regulator genes including cyclinD1 and cdc2 (refs 4 , 5 , 6 , 7 ). In line with this, c-Jun −/− mouse embryonic fibroblasts display severe proliferation defects and deficiency in cell cycle re-entry after serum withdrawal [4] , [8] , [9] . c-Jun also has been demonstrated to be crucial for Ras-driven transformation, as c-Jun knockout mouse embryonic fibroblasts were refractory to the effects of oncogenic Ras [10] . c-Jun responds to growth factor stimulation via extracellular signal-regulated kinase (ERK) as well as cellular stress via the JNK pathway, and mediates diverse cellular responses ranging from proliferation, migration and differentiation to tumorigenesis and cellular apoptosis [4] , [11] , [12] . The activation of c-Jun via JNK has been well characterized [13] , [14] ; however, the molecular mechanism connecting c-Jun and active Ras–Raf–MEK–ERK signalling, potentially crucial to its role in tumourigenesis, remains incomplete. We previously described a novel c-Jun co-activator, RING domain AP-1 co-activator 1 (RACO-1), a RING domain-containing E3 ubiquitin ligase, which is stabilized by growth factor signalling. RACO-1 stability is regulated by a ubiquitin switch between Lys48 (K48)- and Lys63 (K63)-linked ubiquitination, controlled by active MEK [15] and by PRMT1-mediated arginine methylation [16] . Methylation of two arginine residues in the N terminus of RACO-1 (R98, 109) stabilizes RACO-1 in a dimeric conformation and is a prerequisite for all known RACO-1 functions [16] . RACO-1 depletion reduces cellular proliferation and downregulates several growth-associated AP-1 target genes, such as cdc2 , cyclinD1 and hb–egf. On the other hand, transgenic overexpression of RACO-1 augments intestinal tumour formation triggered by aberrant Wnt signalling and cooperates with oncogenic Ras in colon epithelial hyperproliferation [15] . These data indicate that RACO-1 forms part of the link between Ras and c-Jun in tumourigenesis. However, the molecular players inducing the ubiquitin switch downstream of MEK to stabilize RACO-1 were not known. In this study, we identify a previously uncharacterized ubiquitin ligase, Tripartite Motif-containing 7 (Trim7), which on Ras–Raf–MEK–ERK pathway activation, is phosphorylated and activated by MSK1. Trim7 in turn ubiquitinates and stabilizes RACO-1, leading to increased c-Jun transcription. These findings delineate the complete pathway by which growth factor signalling stimulates c-Jun function, and provide further evidence for the importance of phosphorylation–ubiquitination crosstalk in fundamental aspects of cell signalling. Underlining the importance of this pathway in vivo , we find that Trim7 cooperates with oncogenic Ras to drive lung tumorigenesis. Identification of Trim7 as a RACO-1 interacting protein The c-Jun co-activator RACO-1 is stabilized by growth factor signalling via MEK, and is therefore a component of the uncharacterized pathway linking Ras signalling with c-Jun/AP-1 transcription [15] . To identify other components of this pathway, we used a biotinylated peptide (163–235) corresponding to the RACO-1 C terminus, encompassing the ubiquitinated residues K195, K223 and K224, in order to find protein interactors likely to affect RACO-1 stability ( Fig. 1a ). RACO-1 (163–235) or the scrambled peptide was incubated with HeLa cell extract, followed by affinity-capture using streptavidin beads. Using mass spectrometry, we identified a previously uncharacterized ubiquitin ligase, Trim7, interacting with RACO-1. The TRIM family of proteins is identified by tripartite motifs, which consist of a RING domain, followed by a B-Box and a coiled-coil domain. The C-terminal end varies between family members and, in the case of Trim7, contains a C-terminal B30.2 (SPRY) domain [17] ( Fig. 1a ). Flag-tagged RACO-1 co-immunoprecipitated with Myc-tagged Trim7, confirming the interaction ( Fig. 1b ). Fine mapping with different deletion constructs encompassing RACO-1 showed that Trim7 interacts specifically with the very C terminus of RACO-1 ( Supplementary Fig. 1a,b ). 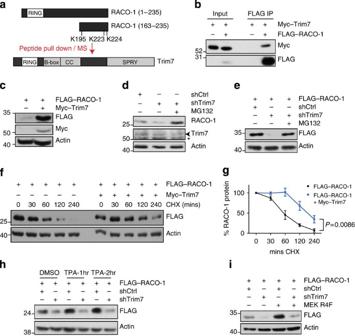Figure 1: Trim7 regulates RACO-1 stability in a MEK-dependent manner. (a) Scheme of mass spectrometry experiment to identify RACO-1 interactors, showing domain structures of RACO-1 and Trim7. RING (zinc finger), B-box, coiled-coil (CC) and SPRY (protein–protein interaction) domains are shown. (b) FLAG–RACO-1 immunoprecipitation from cells transfected with Myc–Trim7 and blotted for Myc and FLAG. (c) Western blots showing the effect of Myc–Trim7 overexpression on FLAG–RACO-1 levels. (d) Western blot showing the effect of Trim7 depletion on endogenous RACO-1 levels in human lung H727 cells, in the presence and absence of proteasome inhibitor (MG132). Arrowhead indicates Trim7 band; asterisk indicates a nonspecific band. (e) Western blots showing the effect of Trim7 depletion on FLAG–RACO-1 levels, in the presence and absence of MG132. (f) Western blots showing the degradation of FLAG–RACO-1 over time in the presence of cycloheximide (CHX), in control cells and cells overexpressing Myc–Trim7. (g) Quantification offand two other similar CHX time course experiments showing RACO-1 stability. Error bars indicate s.e.m.P=0.0086 (Student’st-test comparing RACO-1 levels at 240 min). (h) Western blot showing RACO-1 levels in control and Trim7-depleted cells after treatment with dimethylsulphoxide (vehicle) or TPA to stimulate MEK signalling. (i) Western blots showing the effect of Trim7 depletion by shRNA in the presence or absence of constitutively active MEK (MEKR4F). Actin is shown as loading control. Experiments were replicated at least three times. Figure 1: Trim7 regulates RACO-1 stability in a MEK-dependent manner. ( a ) Scheme of mass spectrometry experiment to identify RACO-1 interactors, showing domain structures of RACO-1 and Trim7. RING (zinc finger), B-box, coiled-coil (CC) and SPRY (protein–protein interaction) domains are shown. ( b ) FLAG–RACO-1 immunoprecipitation from cells transfected with Myc–Trim7 and blotted for Myc and FLAG. ( c ) Western blots showing the effect of Myc–Trim7 overexpression on FLAG–RACO-1 levels. ( d ) Western blot showing the effect of Trim7 depletion on endogenous RACO-1 levels in human lung H727 cells, in the presence and absence of proteasome inhibitor (MG132). Arrowhead indicates Trim7 band; asterisk indicates a nonspecific band. ( e ) Western blots showing the effect of Trim7 depletion on FLAG–RACO-1 levels, in the presence and absence of MG132. ( f ) Western blots showing the degradation of FLAG–RACO-1 over time in the presence of cycloheximide (CHX), in control cells and cells overexpressing Myc–Trim7. ( g ) Quantification of f and two other similar CHX time course experiments showing RACO-1 stability. Error bars indicate s.e.m. P =0.0086 (Student’s t -test comparing RACO-1 levels at 240 min). ( h ) Western blot showing RACO-1 levels in control and Trim7-depleted cells after treatment with dimethylsulphoxide (vehicle) or TPA to stimulate MEK signalling. ( i ) Western blots showing the effect of Trim7 depletion by shRNA in the presence or absence of constitutively active MEK (MEK R4F ). Actin is shown as loading control. Experiments were replicated at least three times. Full size image Next, we investigated the effect of Trim7 on RACO-1 stability. RACO-1 protein is highly unstable in unstimulated conditions, since it is subject to autoubiquitination with K48-linked ubiquitin via its own RING domain and degradation by the proteasome [15] . However, overexpression of Myc–Trim7 in 293T cells greatly increased RACO-1 protein levels ( Fig. 1c ). Conversely, knocking down Trim7 decreased levels of endogenous RACO-1 in the H727 human lung adenocarcinoma cell line. This decrease occurred through proteasome-mediated degradation, as inhibiting the proteasome restored RACO-1 protein levels ( Fig. 1d ). Similar results were obtained with ectopically expressed FLAG-tagged RACO-1, and with two independent trim7 siRNAs ( Fig. 1e and Supplementary Fig. 1c ). Moreover, Trim7 knockdown in H727 cells had no significant effect on RACO-1 mRNA measured by quantitative reverse transcription–PCR (qRT–PCR; Supplementary Fig. 1d ), excluding an effect of Trim7 on RACO-1 transcription. To determine whether Trim7 affects RACO-1 protein stability, we performed a time course experiment to monitor FLAG–RACO-1 degradation in the presence of cycloheximide to inhibit protein synthesis. Overexpression of Myc–Trim7 significantly slowed the degradation of RACO-1 ( Fig. 1f,g ), while knockdown of Trim7 accelerated degradation of the protein ( Supplementary Fig. 1e,f ). Together with the results above, these findings demonstrate that Trim7 stabilizes the RACO-1 protein. Our previous results showed that RACO-1 stability is regulated by MEK–ERK signalling, and the effect of RACO-1 on c-Jun is independent of JNK phosphorylation [15] . In line with this, stimulation of JNK by anisomycin does not increase RACO-1 levels ( Supplementary Fig. 1g ). To test whether Trim7-mediated stabilization of RACO-1 is under the control of the MEK–ERK pathway, Trim7 was knocked down by short hairpin RNA (shRNA) and the cells were treated with phorbol ester (12-O-tetradecanoyl phorbol 13-acetate, TPA), which activates the MEK–ERK pathway. TPA treatment increased RACO-1 protein levels, but failed to do so in Trim7 -depleted samples ( Fig. 1h ). As TPA is known to activate other signalling pathways in addition to MEK–ERK signalling, we used a constitutively active MEK1 (MEK R4F ) to activate the MEK–ERK pathway specifically. MEK R4F increased RACO-1 protein levels in control cells; however, this effect was significantly reduced when Trim7 was knocked down ( Fig. 1i ). These results imply that RACO-1 stabilization by MEK–ERK signalling requires Trim7. Trim7 directly ubiquitinates RACO-1 using K63-linked chains To investigate the mechanistic basis of RACO-1 stabilization by Trim7, 293T cells were transfected with His-ubiquitin and RACO-1 with or without Trim7. In vivo ubiquitination assay using Ni 2+ -NTA pulldown of ubiquitinated proteins showed that Trim7 stimulates RACO-1 ubiquitination ( Fig. 2a ). Next, we used two ubiquitin mutants, K48R and K63R, to identify the chain linkage of ubiquitinated RACO-1. Trim7 stimulated efficient ubiquitination of RACO-1 using K48R ubiquitin; however, ubiquitination was significantly reduced when K63R-mutant ubiquitin was used. Thus, Trim7 promotes RACO-1 ubiquitination with K63-linked ubiquitin chains ( Fig. 2b ). Trim7 is predicted to be a ubiquitin ligase, as it contains a RING domain; however, this has not been experimentally validated. To test whether the RING domain of Trim7 is important for RACO-1 ubiquitination, we mutated Cys29 and Cys32 to alanine (C29,32A), which destroys the integrity of the RING domain. In addition, we mutated a conserved tryptophan residue (Trp57) to alanine (W57A), which is important for the interaction of the RING domain with ubiquitin-conjugating enzymes (E2s) [18] . Both the mutant Trim7 proteins failed to stabilize RACO-1 ( Fig. 2c ). In vivo ubiquitination assay using wild-type (WT) or RING mutant Trim7 also demonstrated the inability of the Trim7 mutants to ubiquitinate RACO-1 ( Fig. 2d ). Interestingly, overexpression of mutant Trim7 reduced FLAG–RACO-1 protein below control levels ( Fig. 2c ), suggesting that the mutant has a dominant-negative effect over the endogenous Trim7. In support of this idea, FLAG-tagged Trim7 was able to pull down Myc-tagged Trim7 by co-immunoprecipitation ( Supplementary Fig. 2a ), suggesting that, in common with other RING E3 ligases, Trim7 may act as a homodimer. 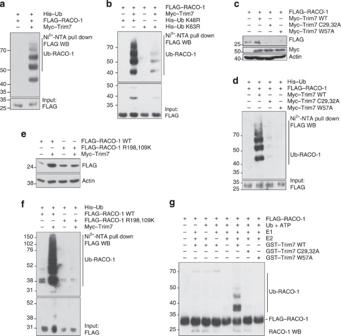Figure 2: Trim7 ubiquitinates RACO-1 through K63 linkage. (a) Ubiquitin pulldown using Ni2+-NTA resin to precipitate ubiquitinated proteins from cells transfected with FLAG–RACO-1 and Myc–Trim7 as indicated. (b) Ubiquitin pulldown as above using K48R or K63R-mutant ubiquitin, which cannot form K48- or K63-linked ubiquitin chains, respectively. (c) Western blots showing FLAG–RACO-1 levels in Trim7-depleted cells reconstituted with WT, RING domain mutant (C29,32A) or E2 interaction mutant (W57A) Trim7. (d) Ubiquitin pulldown from cells expressing the above Trim7 mutants. (e) Western blots showing FLAG–RACO-1 and FLAG–RACO-1 R198,109K levels in the presence or absence of Trim7 overexpression. The R198,109K mutation disrupts the PRMT1 methylation sites and prevents RACO-1 dimerization. (f) Ubiquitin pulldown from cells expressing FLAG–RACO-1 or FLAG–RACO-1 R198,109K and Myc–Trim7 as indicated. (g)In vitroubiquitination assay using the indicated components together with immunoprecipitated FLAG–RACO-1 and purified recombinant GST–Trim7 WT, GST–Trim7 C29,32A or GST–Trim7 W57A. Experiments were replicated at least three times. Figure 2: Trim7 ubiquitinates RACO-1 through K63 linkage. ( a ) Ubiquitin pulldown using Ni 2+ -NTA resin to precipitate ubiquitinated proteins from cells transfected with FLAG–RACO-1 and Myc–Trim7 as indicated. ( b ) Ubiquitin pulldown as above using K48R or K63R-mutant ubiquitin, which cannot form K48- or K63-linked ubiquitin chains, respectively. ( c ) Western blots showing FLAG–RACO-1 levels in Trim7-depleted cells reconstituted with WT, RING domain mutant (C29,32A) or E2 interaction mutant (W57A) Trim7. ( d ) Ubiquitin pulldown from cells expressing the above Trim7 mutants. ( e ) Western blots showing FLAG–RACO-1 and FLAG–RACO-1 R198,109K levels in the presence or absence of Trim7 overexpression. The R198,109K mutation disrupts the PRMT1 methylation sites and prevents RACO-1 dimerization. ( f ) Ubiquitin pulldown from cells expressing FLAG–RACO-1 or FLAG–RACO-1 R198,109K and Myc–Trim7 as indicated. ( g ) In vitro ubiquitination assay using the indicated components together with immunoprecipitated FLAG–RACO-1 and purified recombinant GST–Trim7 WT, GST–Trim7 C29,32A or GST–Trim7 W57A. Experiments were replicated at least three times. Full size image Previously, we have shown that active RACO-1 is a homodimer and PRMT1-mediated methylation of RACO-1 is a prerequisite for efficient dimer formation [16] . In order to identify whether Trim7 preferentially ubiquitinates dimeric RACO-1, we used a mutant RACO-1 lacking two arginines that are targets for PRMT1-mediated methylation (RACO-1 R98,109K) that is, therefore, compromised in dimerization ability. Overexpression of Trim7 did not stabilize RACO-1 R98,109K ( Fig. 2e ), and in vivo ubiquitination assay revealed that Trim7 was unable to stimulate ubiquitination of this mutant protein ( Fig. 2f ), suggesting that dimeric RACO-1 is the optimal substrate for Trim7. Next, we wanted to test whether Trim7 directly ubiquitinates RACO-1. Ectopically expressed FLAG–RACO-1 was immunoprecipitated from 293T cells and was used as a substrate for in vitro ubiquitination assay ( Fig. 2g ). Recombinant GST (glutathione S -transferase)-tagged Trim7 ubiquitinated RACO-1 only when all the purified components of the ubiquitination cascade (ubiquitin, ATP, E1, E2 and E3 ligases) were present. Moreover, the C29,32A and W57A mutants of Trim7 did not ubiquitinate RACO-1 ( Fig. 2g ), implying that RACO-1 ubiquitination requires a functional Trim7 RING domain. Taken together, these data suggest that Trim7 directly ubiquitinates RACO-1. RACO-1 stabilization by MEK requires MSK1 activity We next investigated the mechanism of Trim7 regulation by growth factor signalling. The requirement of Trim7 for RACO-1 stabilization by MEK R4F ( Fig. 1i ) suggested that the Trim7-regulatory activity is downstream of MEK. Knocking down ERK1/2 in 293T cells reduced RACO-1 levels, suggesting that Trim7 is under the control of ERK activity ( Supplementary Fig. 2b ). To test whether ERK directly phosphorylates Trim7, we carried out an in vitro kinase assay. Recombinant ERK efficiently phosphorylated Elk-1, a canonical ERK substrate, but did not phosphorylate Trim7 ( Supplementary Fig. 2c ). Mitogen and stress-activated protein kinase (MSK) and 90-kDa ribosomal S6 kinase (RSK) kinases mediate signal transduction downstream of MAPK signalling. Both the kinases are directly phosphorylated and activated by ERK kinases [19] , [20] . In addition, MSK1 has been shown to induce immediate early gene expression on Ras activation, via the nucleosomal response [21] , [22] , [23] . We therefore tested the effect of two MSK inhibitors, H-89 and Ro-31–8220, as well as RSK inhibitor II, on RACO-1 stability ( Fig. 3a ). Both MSK inhibitors destabilized RACO-1, while RSK inhibitor II had no effect on RACO-1 protein levels, suggesting that MSK is probably responsible for transducing the signals from active MEK–ERK signalling towards RACO-1 ( Fig. 3b ). The destabilization of RACO-1 by Ro-31–8220 was proteasome-dependent, as adding proteasome inhibitor reverted this effect ( Fig. 3c ). Inhibition of the MEK–ERK pathway in H727 cells with the MEK inhibitor U0126 and the MSK inhibitor Ro-31–8220 decreased endogenous RACO-1 protein levels to a similar extent ( Fig. 3d ). 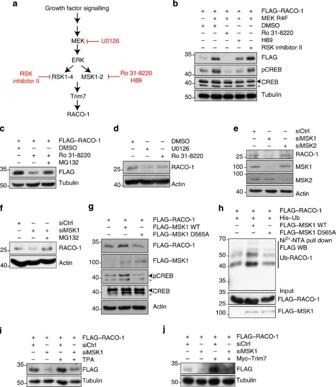Figure 3: RACO-1 stabilization by MEK requires MSK1. (a) Simplified scheme of the MEK signalling pathway showing possible downstream effectors of Trim7 and RACO-1 regulation. Kinase inhibitors are shown in red. (b) Western blots showing the effect of the indicated kinase inhibitors on MEKR4F-induced FLAG–RACO-1 protein levels. Phosphorylated CREB (pCREB) is shown as a control for MSK inhibition. Tubulin is shown as loading control. Arrowhead indicates CREB band; asterisk indicates a nonspecific band. (c) Western blots showing the effect of the MSK inhibitor Ro-31–8220 on FLAG–RACO-1 levels in the presence and absence of MG132. (d) Western blot showing the effect of the indicated inhibitors on endogenous RACO-1 levels in H727 cells. (e) siRNA-mediated depletion of MSK1 and MSK2 in H727 cells, showing the effect on endogenous RACO-1 levels. (f) Western blots showing the effect of MSK1 depletion on endogenous RACO-1 levels in H727 cells, in the presence and absence of MG132. (g) Western blot showing FLAG–RACO-1 levels in cells transfected with MSK1 or the catalytically impaired MSK1 mutant D565A. pCREB is shown as a control for MSK1 activity. Arrowhead indicates CREB/pCREB band; asterisk indicates a nonspecific band. (h) Ubiquitin pulldown from cells expressing MSK1 or D565A mutant MSK1, showing ubiquitinated FLAG–RACO-1. (i) Western blots showing the effect of MSK1 depletion by siRNA on FLAG–RACO-1 levels in the presence or absence of TPA. (j) Western blots showing the effect of MSK1 depletion by siRNA on FLAG–RACO-1 levels in the presence or absence of Myc–Trim7 overexpression. Experiments were replicated at least three times. Figure 3: RACO-1 stabilization by MEK requires MSK1. ( a ) Simplified scheme of the MEK signalling pathway showing possible downstream effectors of Trim7 and RACO-1 regulation. Kinase inhibitors are shown in red. ( b ) Western blots showing the effect of the indicated kinase inhibitors on MEK R4F -induced FLAG–RACO-1 protein levels. Phosphorylated CREB (pCREB) is shown as a control for MSK inhibition. Tubulin is shown as loading control. Arrowhead indicates CREB band; asterisk indicates a nonspecific band. ( c ) Western blots showing the effect of the MSK inhibitor Ro-31–8220 on FLAG–RACO-1 levels in the presence and absence of MG132. ( d ) Western blot showing the effect of the indicated inhibitors on endogenous RACO-1 levels in H727 cells. ( e ) siRNA-mediated depletion of MSK1 and MSK2 in H727 cells, showing the effect on endogenous RACO-1 levels. ( f ) Western blots showing the effect of MSK1 depletion on endogenous RACO-1 levels in H727 cells, in the presence and absence of MG132. ( g ) Western blot showing FLAG–RACO-1 levels in cells transfected with MSK1 or the catalytically impaired MSK1 mutant D565A. pCREB is shown as a control for MSK1 activity. Arrowhead indicates CREB/pCREB band; asterisk indicates a nonspecific band. ( h ) Ubiquitin pulldown from cells expressing MSK1 or D565A mutant MSK1, showing ubiquitinated FLAG–RACO-1. ( i ) Western blots showing the effect of MSK1 depletion by siRNA on FLAG–RACO-1 levels in the presence or absence of TPA. ( j ) Western blots showing the effect of MSK1 depletion by siRNA on FLAG–RACO-1 levels in the presence or absence of Myc–Trim7 overexpression. Experiments were replicated at least three times. Full size image The MSK protein kinase family consists of two members, MSK1 and MSK2. To determine whether MSK1 or MSK2 is responsible for RACO-1 stabilization, we depleted each of these proteins individually by siRNA. Depletion of MSK1, but not MSK2, reduced endogenous RACO-1 protein levels, and this effect was rescued by proteasome inhibitor, suggesting that MSK1 is required for the stabilization of endogenous RACO-1 ( Fig. 3e,f ). In support of this, overexpression of WT MSK1 increased RACO-1 protein levels, but a catalytically dead MSK1 protein (MSK1 D565A (ref. 20 )) did not ( Fig. 3g ). In vivo ubiquitination assay also confirmed this conclusion, as overexpression of WT MSK1 increased RACO-1 ubiquitination, while MSK1 D565A had no effect ( Fig. 3h ). MSK1 was required for RACO-1 protein stabilization by TPA ( Fig. 3i ). Similarly, MSK1 was also required for efficient RACO-1 stabilization by Trim7 overexpression, suggesting that RACO-1 stabilization by MEK–ERK signalling requires MSK1 ( Fig. 3j ). MSK1 directly phosphorylates Trim7 To investigate the mechanism of MSK1-mediated signal transduction resulting in RACO-1 stabilization, we tested whether MSK1 directly phosphorylates Trim7. Wild-type MSK1 and the kinase-dead MSK1 D565A mutant were overexpressed in 293T cells, immunoprecipitated, and used for in vitro kinase assay using radioactive γ 32 P-ATP. Wild-type MSK1 specifically phosphorylated recombinant GST–Trim7, while MSK1 D565A did not, suggesting that MSK1 directly phosphorylates Trim7 ( Fig. 4a ). MSK kinases phosphorylate serine residues within the consensus sequence R/KxRxxS or RRxS. Analysis of the Trim7 amino-acid sequence revealed a consensus phosphorylation site, Ser107, for the MSK kinases ( Supplementary Fig. 2d ). Mutation of the S107 site on Trim7 abolished this phosphorylation ( Fig. 4b ), confirming S107 as the MSK1 phosphorylation site on Trim7. 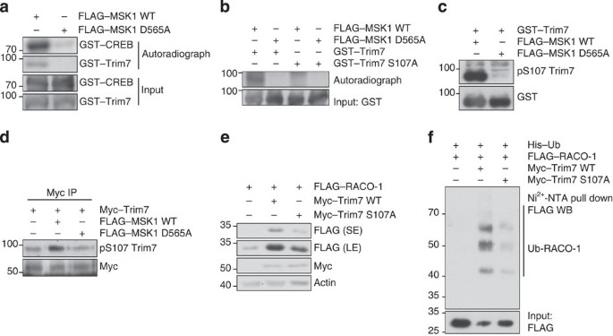Figure 4: MSK1 directly phosphorylates Trim7 and regulates RACO-1 stability. (a)In vitrokinase assay using recombinant GST–Trim7 as a substrate for phosphorylation by FLAG–MSK1. GST–CREB and MSK1 D565A are shown as positive and negative controls, respectively. (b)In vitrokinase assay using recombinant GST–Trim7 or mutant GST–Trim7 S107A as a substrate for phosphorylation by FLAG–MSK1. (c) Western blot showing Trim7 phosphorylation at S107, using pS107 Trim7 antibody. (d) Myc–Trim7 immunoprecipitation from cells transfected with FLAG–MSK1 or FLAG–MSK1 D565A, showing Trim7 phosphorylation at S107. (e) Western blot showing FLAG–RACO-1 levels in cells transfected with Myc–Trim7 or mutant Myc–Trim7 S107A. LE, long exposure; SE, short exposure. (f) Ubiquitin pulldown from cells expressing Myc–Trim7 or mutant Myc–Trim7 S107A, showing ubiquitinated FLAG–RACO-1. Note that the amount of lysate was adjusted to account for the stabilization of RACO-1 in Trim7-overexpressing cells, and so input levels do not reflect the amount of RACO-1 protein in cells. Experiments were replicated at least three times. Figure 4: MSK1 directly phosphorylates Trim7 and regulates RACO-1 stability. ( a ) In vitro kinase assay using recombinant GST–Trim7 as a substrate for phosphorylation by FLAG–MSK1. GST–CREB and MSK1 D565A are shown as positive and negative controls, respectively. ( b ) In vitro kinase assay using recombinant GST–Trim7 or mutant GST–Trim7 S107A as a substrate for phosphorylation by FLAG–MSK1. ( c ) Western blot showing Trim7 phosphorylation at S107, using pS107 Trim7 antibody. ( d ) Myc–Trim7 immunoprecipitation from cells transfected with FLAG–MSK1 or FLAG–MSK1 D565A, showing Trim7 phosphorylation at S107. ( e ) Western blot showing FLAG–RACO-1 levels in cells transfected with Myc–Trim7 or mutant Myc–Trim7 S107A. LE, long exposure; SE, short exposure. ( f ) Ubiquitin pulldown from cells expressing Myc–Trim7 or mutant Myc–Trim7 S107A, showing ubiquitinated FLAG–RACO-1. Note that the amount of lysate was adjusted to account for the stabilization of RACO-1 in Trim7-overexpressing cells, and so input levels do not reflect the amount of RACO-1 protein in cells. Experiments were replicated at least three times. Full size image We generated an antibody specifically recognizing phosphorylated serine 107 of Trim7 to further investigate Trim7 regulation. The pS107–Trim7 antibody detected Trim7 phosphorylated with WT MSK1, but not the unphosphorylated Trim7, demonstrating the specificity of the antibody ( Fig. 4c ). Ectopic MSK1 expression increased Trim7 phosphorylation at S107, validating that this modification occurs in vivo ( Fig. 4d ). Mutation of Trim7 S107 to alanine inhibited the stabilization of RACO-1, suggesting that phosphorylation of this site is required for stimulation of Trim7 activity ( Fig. 4e ). Consistent with this, Trim7 S107A was less able to ubiquitinate RACO-1 ( Fig. 4f ). To determine whether phosphorylation of Trim7 S107A affected its interaction with RACO-1, we performed co-immunoprecipitation experiments. Neither activation nor inhibition of MEK signalling (by TPA or U0126, respectively) nor mutation of the S107 phosphorylation site on Trim7 affected its interaction with RACO-1 ( Supplementary Fig. 3a,b ), suggesting that MEK-induced phosphorylation of Trim7 promotes its E3 ligase activity by increasing the efficiency of ubiquitin transfer rather than enhancing the interaction with RACO-1. Taken together, our data suggest that on activation of the Ras–Raf–MEK–ERK pathway, MSK1 phosphorylates Trim7 on serine 107 and stimulates its E3 ligase activity towards RACO-1, resulting in RACO-1 stabilization. Trim7 promotes oncogenic Ras-mediated lung adenocarcinoma Adenocarcinoma, a form of non-small cell lung cancer, is the most common type of lung cancer in humans. K-Ras mutations are commonly found in non-small cell lung cancers and are believed to play a key role in this malignancy. Data from The Cancer Genome Atlas indicate that Trim7 is altered in 5% of human lung adenocarcinomas, most frequently by overexpression ( Supplementary Fig. 4a ). Moreover, amplified or overexpressed RACO-1, present in 8% of these tumours, does not overlap with Trim7 alteration, and there is also a tendency towards mutual exclusivity with K-Ras mutations ( Supplementary Fig. 4a ) [24] , [25] , in support of K-Ras, Trim7 and RACO-1 being in the same pathway. Thus, we used a Ras-driven lung cancer model [26] , [27] to test the significance of the Trim7/RACO-1 axis in tumourigenesis. In this mouse model, Cre-mediated recombination induces the expression of oncogenic K-Ras G12D (ref. 27 ). The transgene expression was activated in the lung by tracheal intubation of mice with Cre-expressing adenovirus ( Adeno-Cre ) [26] . For transgenic overexpression of Trim7, we targeted a Cre-inducible human Trim7 transgene to the Rosa26 locus. The expression of the transgene is dependent on Cre recombinase-mediated excision of a STOP cassette ( Rosa26-loxSTOPlox-Trim7-IRES-GFP or R26Trim7 ). The ‘ KT ’ model combined inducible K-Ras G12D expression with transgenic Trim7 and green fluorescent protein (GFP) expression from the Rosa26 promoter ( LSL - K-Ras G12D ; R26-LSL-Trim7-IRES-GFP; plus Adeno-Cre ; Fig. 5a ). Total lung extracts from either K-Ras G12D or KT mice were used to isolate RNA and protein. Quantitative RT–PCR showed the expression of the Trim7 transgene in the lungs of KT mice ( Fig. 5b ). Western blot analysis of the proteins showed a significant stabilization of RACO-1 in KT mice compared with K-Ras G12D mice ( Fig. 5c ). 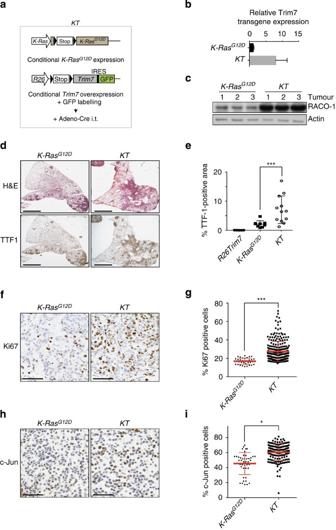Figure 5: RACO-1 and Trim7 cooperate with K-RasG12Dto drive lung tumorigenesis. (a) Scheme ofKTmouse model. i.t., intratracheal. (b) Quantitative PCR showing expression of the Trim7 transgene inKTmouse lung tissue. Error bars indicate s.d.n=3 tumours per genotype. (c) Western blot showing RACO-1 protein levels inKTmouse lung tissue. (d) Haematoxylin and eosin (H&E) stain and TTF-1 immunohistochemistry on whole-lung sections fromKTandK-RasG12Dmice 12 weeks after Cre induction ( × 1.25 magnification). Scale bar, 2 mm. (e) Quantification of the percentage of total lung area stained with TTF-1 in mice of the indicated genotypes. Each data point represents a whole-lung section from one mouse.n=5R26Trim7, 9K-RasG12Dand 12KTmice. (f,g) Staining ( × 40 magnification;f) and quantification (g) of Ki67-positive cells in lung tumours from mice of the indicated genotypes. Each data point represents one tumour. All tumours from one lung section per mouse were analysed (five mice per genotype).n=36K-RasG12Dand 243KTtumours. (h,i) Staining ( × 40 magnification;h) and quantification (i) of c-Jun-positive cells in lung tumours from mice of the indicated genotypes. Each data point represents one tumour. All tumours from one lung section per mouse were analysed (five mice per genotype).n=43K-RasG12Dand 151KTtumours. *P=0.02, ***P<0.001 (Student’st-test). Error bars ine,g,iindicate mean±s.e.m. Scale bars inf,h, 100 μm. Figure 5: RACO-1 and Trim7 cooperate with K-Ras G12D to drive lung tumorigenesis. ( a ) Scheme of K T mouse model. i.t., intratracheal. ( b ) Quantitative PCR showing expression of the Trim7 transgene in KT mouse lung tissue. Error bars indicate s.d. n =3 tumours per genotype. ( c ) Western blot showing RACO-1 protein levels in KT mouse lung tissue. ( d ) Haematoxylin and eosin (H&E) stain and TTF-1 immunohistochemistry on whole-lung sections from KT and K-Ras G12D mice 12 weeks after Cre induction ( × 1.25 magnification). Scale bar, 2 mm. ( e ) Quantification of the percentage of total lung area stained with TTF-1 in mice of the indicated genotypes. Each data point represents a whole-lung section from one mouse. n =5 R26Trim7 , 9 K-Ras G12D and 12 KT mice. ( f , g ) Staining ( × 40 magnification; f ) and quantification ( g ) of Ki67-positive cells in lung tumours from mice of the indicated genotypes. Each data point represents one tumour. All tumours from one lung section per mouse were analysed (five mice per genotype). n =36 K-Ras G12D and 243 KT tumours. ( h , i ) Staining ( × 40 magnification; h ) and quantification ( i ) of c-Jun-positive cells in lung tumours from mice of the indicated genotypes. Each data point represents one tumour. All tumours from one lung section per mouse were analysed (five mice per genotype). n =43 K-Ras G12D and 151 KT tumours. * P =0.02, *** P <0.001 (Student’s t -test). Error bars in e , g , i indicate mean±s.e.m. Scale bars in f , h , 100 μm. Full size image As expected, expression of oncogenic K-Ras G12D alone resulted in formation of hyperplastic lesions and adenomas in the lungs that stain positive for TTF-1 ( Fig. 5d ). TTF-1 is frequently overexpressed in lung adenocarcinoma, and routinely used as a marker for these tumours [28] , [29] . Quantification of the TTF-1-positive transformed area of the lungs from K-Ras G12D and KT mice showed a significant increase in tumour burden in KT mice ( Fig. 5d,e ), whereas transgenic overexpression of Trim7 alone did not result in any TTF-1-positive lesions ( Fig. 5e ). Detailed analysis of the tumours was carried out by immunohistochemical staining of the lung. Tumours from both mouse genotypes were positive for TTF-1 and surfactant protein C, implying that they are adenocarcinomas ( Supplementary Fig. 4b ). KT tumours had significantly increased cellular proliferation compared with K-Ras G12D tumours, as judged by quantification of Ki67-positive cells ( Fig. 5f,g ). Quantification of the percentage of c-Jun-positive cells per tumour showed a mild but significant increase in KT mice compared with K-Ras G12D mice ( Fig. 5h,i ). Taken together, these data demonstrate that Trim7 cooperates with oncogenic Ras in lung adenocarcinoma formation. Trim7 depletion restrains tumour cell proliferation RACO-1 acts as a transcriptional co-activator of c-Jun and reduced RACO-1 level leads to a reduction in c-Jun transcriptional activity [15] , [16] . A luciferase assay using a stably integrated chromosomal AP-1 reporter construct (collagenase–luciferase) showed a similar decrease in gene expression when either Trim7 or RACO-1 were depleted with shRNA, consistent with Trim7 regulating the transcription of c-Jun/AP-1 target genes via RACO-1 ( Fig. 6a ). 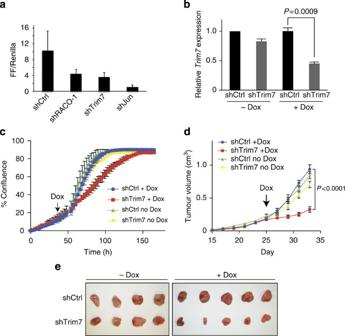Figure 6: Trim7 depletion in established tumours reduces tumour growth. (a) Luciferase assay in HeLa cells containing a stably integrated chromosomal collagenase–luciferase reporter as a read-out for AP-1 transcription. Error bars indicate s.d. (b) Quantitative PCR showing the level of Trim7 mRNA expression in H727 cells stably carrying doxycycline (Dox)-inducible shRNA constructs. Error bars indicate s.d. (c) Time course showing proliferation of cells inbin vitrowith and without addition of Dox to induce expression of the indicated shRNA. % Confluence was measured automatically by Incucyte time lapse microscopy and used as a read-out for cell proliferation. Error bars indicate s.d. (d) Time course showing growth of xenograft tumours from NOD-SCID mice following subcutaneous injection with H727 cells stably carrying Dox-inducible shRNA. Tumours were allowed to establish for 25 days and then animals were treated daily with Dox to induce Trim7 knockdown in the xenograft. The growth of similar xenografts in mice not treated with Dox is shown as a control. Tumours were measured with calipers every 2 days.n=5 mice (+Dox) and 4 mice (−Dox). Error bars indicate s.e.m.P<0.0001 at 33 days (Student’st-test). (e) Xenograft tumours from the experiment indshown at experimental end point. Figure 6: Trim7 depletion in established tumours reduces tumour growth. ( a ) Luciferase assay in HeLa cells containing a stably integrated chromosomal collagenase–luciferase reporter as a read-out for AP-1 transcription. Error bars indicate s.d. ( b ) Quantitative PCR showing the level of Trim7 mRNA expression in H727 cells stably carrying doxycycline (Dox)-inducible shRNA constructs. Error bars indicate s.d. ( c ) Time course showing proliferation of cells in b in vitro with and without addition of Dox to induce expression of the indicated shRNA. % Confluence was measured automatically by Incucyte time lapse microscopy and used as a read-out for cell proliferation. Error bars indicate s.d. ( d ) Time course showing growth of xenograft tumours from NOD-SCID mice following subcutaneous injection with H727 cells stably carrying Dox-inducible shRNA. Tumours were allowed to establish for 25 days and then animals were treated daily with Dox to induce Trim7 knockdown in the xenograft. The growth of similar xenografts in mice not treated with Dox is shown as a control. Tumours were measured with calipers every 2 days. n =5 mice (+Dox) and 4 mice (−Dox). Error bars indicate s.e.m. P <0.0001 at 33 days (Student’s t -test). ( e ) Xenograft tumours from the experiment in d shown at experimental end point. Full size image In human lung adenocarcinoma, oncogenic Ras mutations are frequently associated with mutations in other tumour suppressors such as p53 (ref. 30 ). Therefore, to test the effects of Trim7 depletion, we used primary murine lung adenocarcinoma cells derived from a K-Ras G12D ; p53 ΔL/ΔL ( KP ) mouse line, which closely resembles human lung adenocarcinoma ( Supplementary Fig. 5a ). We generated KP cells stably expressing two different shRNAs against Trim7. Trim7 depletion suppressed the proliferation of KP cells, and the reduction in proliferation correlated with the extent of Trim7 knockdown in the two cell lines ( Supplementary Fig. 5b,c ). Trim7 depletion in KP cells with the most efficient knockdown construct (shTrim7-2) resulted in a reduced level of RACO-1 ( Supplementary Fig. 5d ) and quantitative RT–PCR analysis revealed that c-Jun target genes were downregulated in Trim7 knockdown cells ( Supplementary Fig. 5e ), supporting the observation that Trim7 regulates c-Jun transactivation function and cellular proliferation. To test the in vivo effect of Trim7 knockdown on KP cells, we subcutaneously injected shControl cells in the left flank and shTrim7-2 cells in the right flank of NOD-SCID mice. Trim7 knockdown resulted in significantly smaller xenograft tumours after 20 days ( Supplementary Fig. 5f,g ). To further test the effect of Trim7 depletion in a clinically relevant scenario, we decided to knock down Trim7 in an already established tumour. To achieve this we generated H727 cell lines expressing a doxycycline-inducible shTrim7 or shControl construct ( Fig. 6b ). We first measured the proliferation of these cell lines in vitro . Cells were plated and allowed to grow for 36 h without doxycycline, at which stage the proliferation of both cell lines was comparable. After 36 h, cells were treated with 2 μg ml −1 doxycycline and their proliferation was monitored for a further 120 h period. On doxycycline treatment, shTrim7-expressing cells showed a significant decrease in proliferation ( Fig. 6c ). Next, we carried out a xenograft experiment with these cell lines. After subcutaneous injection of untreated shControl and shTrim7 cells into NOD-SCID mice as before, xenografts were allowed to grow to a palpable tumour mass, and then mice were given doxycycline every day to induce and maintain the expression of the shRNA. In control mice that did not receive doxycycline treatment, tumours grew equally ( Fig. 6d,e ). In the cohort that received doxycycline treatment, shTrim7-expressing tumours grew significantly slower than the control tumours ( Fig. 6d,e ). This experiment demonstrates that depletion of Trim7 in an established tumour can slow tumour cell proliferation. We conclude that Trim7 functions to stabilize RACO-1 and stimulate c-Jun-mediated gene expression and cellular proliferation, and is required for efficient tumour growth driven by oncogenic Ras. More than 25 years ago AP-1 was identified as an activity that bound to DNA elements in the promoters of the metallothionein and collagenase genes [31] , [32] . The tumour promoter TPA dramatically increases transcription of these genes in an AP-1-dependent manner. The classical Jun/Fos AP-1-binding site, TGACTCA, was identified as the element that mediates TPA induction of the metallothionein and collagenase genes, and is therefore known as the TPA response element. TPA strongly activates the MEK/ERK MAP kinase pathway, but is only a weak activator of JNK signalling and c-Jun N-terminal phosphorylation [33] . However, while JNK-mediated c-Jun phosphorylation is a well-established means of stimulating c-Jun/AP-1 activity, the precise molecular connection between c-Jun and growth factor signalling that is independent of N-terminal phosphorylation has been enigmatic. Our previous work demonstrated that RACO-1 functions as a molecular link between Ras signalling and c-Jun activity [15] . RACO-1 acts as a transcriptional co-activator of c-Jun and stimulates expression of target genes required for cellular proliferation, such as cyclinD1 , cdc2 and hb–egf . RACO-1 stability plays a central role in the regulation of Ras-c-Jun crosstalk. On activation of growth factor signalling, the ubiquitination of RACO-1 shifts from degradative K48-linked autoubiquitination to a nondegradative K63-linked ubiquitination, thereby increasing RACO-1 protein levels and AP-1 activity. In addition, PRMT1-mediated methylation is required for RACO-1 to form a stable dimer, which is responsive to MEK–ERK signalling and can interact with c-Jun. Here we have identified the E3 ubiquitin ligase Trim7 as another important regulator of Ras-c-Jun crosstalk, responsible for MEK-driven stabilization of RACO-1 ( Fig. 7 ). 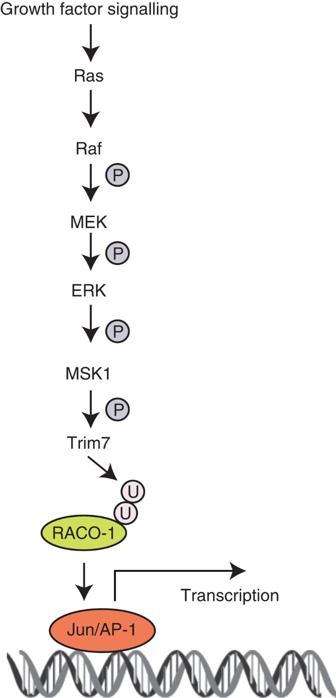Figure 7: Schematic model of the pathway linking Ras with c-Jun/AP-1. A phosphorylation/ubiquitination cascade via MSK1, Trim7 and RACO-1 links growth factor signalling to c-Jun/AP-1 activation. Figure 7: Schematic model of the pathway linking Ras with c-Jun/AP-1. A phosphorylation/ubiquitination cascade via MSK1, Trim7 and RACO-1 links growth factor signalling to c-Jun/AP-1 activation. Full size image Trim family proteins are involved in a broad range of biological processes, and their alterations are associated with diverse pathological conditions, such as developmental disorders, neurodegenerative diseases, viral infections and cancer [34] , [35] , [36] . Trim7 was first identified as glycogenin interacting protein and shown to be important in glycogen biosynthesis [37] . Although ubiquitin ligase activity has been predicted for Trim7 because of the presence of the RING domain, no experimental validation has been carried out. Our data suggest that Trim7 has ubiquitin ligase activity towards RACO-1. On MEK–ERK activation, the ERK downstream kinase MSK1 is activated through phosphorylation, and active MSK1 phosphorylates Trim7, thereby stimulating its activity towards RACO-1. As with many other enzymes, activation by phosphorylation is common among E3 ubiquitin ligases; for example, the regulation of c-Jun turnover through JNK-dependent phosphorylation of the E3 ligase Itch [38] , [39] . The crosstalk between different post-translational modifications has become a recurring theme in biology [40] , and many signalling pathways, including the Ras–Raf–MEK–ERK pathway, are subject to multiple protein modifications including farnesylation [3] , phosphorylation [3] , ubiquitination [41] , [42] , sumoylation [43] and methylation [44] , [45] , among others. This enables the pathway to be responsive to different signal inputs with tighter multilayered regulation. Our study adds to the growing body of data showing that phosphorylation and ubiquitination not only cooperate via priming or competing modifications on the same protein, but also contribute as integral components of signal transmission cascades [40] , [41] , [46] . A significant amount of research has been carried out to develop inhibitors of the Ras signalling pathway for therapeutic intervention in human malignancies. It is becoming increasingly apparent that monotherapy targeting a single kinase is only transiently effective, as the cells become resistant to the inhibitor via various mechanisms, as in the case of the B-Raf inhibitor vemurafenib [47] , [48] , [49] , [50] , [51] . Combined inhibition of B-Raf and MEK has shown promising results and has now been approved for treatment of B-Raf-V600E metastatic melanoma. However, the long-term efficacy of this treatment has been limited by emergence of resistance through mutation in MEK and copy number gain in B-RAF-V600E (ref. 52 ). Targeting effectors downstream of ERK is a promising approach, which could improve efficacy and reduce toxicity [53] , [54] . Our data show that knocking down Trim7 in primary KP lung tumour cells reduced cell proliferation, and significantly decreased tumour growth in xenograft experiments. Moreover, depletion of Trim7 in an established xenograft tumour also reduced tumour growth, supporting the idea that therapeutic intervention in the MSK1/Trim7/RACO-1 signalling pathway is potentially promising. Cell lines and antibodies Human embryonic kidney (HEK) 293T cells, human lung adenocarcinoma H727 cells and primary murine lung adenocarcinoma cells were maintained in Dulbecco’s modified Eagle’s medium (DMEM) supplemented with 10% fetal calf serum. HEK293T and H727 cells were obtained from Cancer Research UK Cell Services. Polyclonal RACO-1 (HPA030098) and Trim7 (HPA039213) antibodies were from Sigma. Antibodies against p-ERK1/2 (9106), total ERK1/2 (9102), pCREB (9191), total CREB (9197), MSK1 (3489) and MSK2 (3679) were from Cell Signaling Technology; Jun (610326) from BD Transduction Laboratories; Flag (A8592) and HA (haemagglutinin; H 6908) from Sigma; β-actin (ab49900), GFP (ab290) from Abcam; and GST (sc-459) from Santa Cruz. Mouse monoclonal antibody against Myc tag was generated in-house. Anti-FLAG horseradish peroxidase (HRP) antibody was used at 1:5,000 dilution and anti-β-actin HRP antibody was used at 1:30,000 dilution. All other antibodies were used at 1:1,000 dilution for western blots. Uncropped scans of western blots are shown in Supplementary Fig. 6 . cDNA constructs and transfections RACO-1 cDNA was cloned in BamHI–EcoRI sites of pCMV2B to generate FLAG–RACO-1, and in HindIII–BamHI sites of pEGFP(C3) to generate GFP–RACO-1. Deletion mutants and point mutants of RACO-1 were generated in the FLAG–RACO-1 construct and verified by sequencing [15] . Human Trim7 isoform 1 cDNA in pDONR vector (Invitrogen) was obtained from Genecopoeia and transferred to N-terminal Myc and GST-tagged pDEST vector (Invitrogen) by LR recombination, as per the manufacturer’s instructions. Site-directed mutagenesis of Trim7 was carried out on Trim7/pDONR and then moved to Myc- or GST-tagged pDEST vector by LR recombination. His-tagged ubiquitin K48R and ubiquitin K63R constructs were a gift from Andreas Hock (University of Marburg, Germany), and MEK1 R4F was a gift from Melanie Cobb (The University of Texas Southwestern Medical Center). Flag-tagged MSK1, MSK1 D565A and GST-tagged CREB were obtained from the MRC Protein Phosphorylation and Ubiquitylation Unit, Dundee. All mutagenic constructs generated were confirmed by sequence analysis. HEK293T and H727 cells were transfected with polyethyleneimine. RNA interference constructs and Lentivirus production siRNA sequences for human Trim7, MSK1 and MSK2 knockdown were designed using Dharmacon siDESIGN centre. Oligonucleotide sequences (sense strand) were: siTrim7 (1): 5′-CGGAAAAGAAGGAGAGCAA-3′; siTrim7 3′ untranslated repeat (2): 5′-GCAUCACGGCUCUCCAGCA-3′; siMSK1 (1): 5′-GCAGAAGAGUUCACAGAAA-3′; siMSK1 (2): 5′-GGAAAUAACAGCUCUGAAA-3′; siMSK2 (1): 5′-CGGCCGAGAUCAUGUGCAA-3′; siMSK2 (2): 5′-GCCGAGAUCAUGUGCAAAA-3′. RISC free siRNA from Dharmacon was used as a control. shRNA sequence for human RACO-1 (5′-tgTGATGGACCGTAGGAAGAAttcaagagaTTCTTCCTACGGTCCATCAttttttc-3′) was cloned into the IRES-GFP lentiviral construct pLentiLox 3.7 (ref. 16 ). shRNA for human c-Jun (SHCLND-NM_002228) and non-targeting shRNA (SHC016) were obtained from Sigma. siTrim7(1) was cloned into pLentiLox 3.7. Hairpin sequence (shown in upper case characters) was: shTrim7- 5′-tgCGGAAAAGAAGGAGAGCAAttcaagagaTTGCTCTCCTTCTTTTCCGttttttc-3′. shRNA against luciferase (5′-tgCGTACGCGGAATACTTCGAttcaagagaTCGAAGTATTCCGCGTACGttttttc-3′) was cloned in pLentiLox 3.7 and used as a control. GIPZ shRNA constructs for mouse Trim7 (shTrim7-1, clone V3LMM_428696: 5′-GAACTTCTTCAGCAATCCT-3′ and shTrim7-2, clone V3LMM_428699: 5′-TGTTGAGTTGCATTGCCCA-3′) and TRIPZ Dox-inducible shRNA constructs for human Trim7 (shTrim7, clone V3THS_351926: 5′-TGAGCTGTCTCCTGGATCT-3′) were obtained from Thermo Scientific. For lentiviral production, low-passage HEK293T was transfected with the respective shRNA construct and the accessory plasmids VSV-G and Δ8.2 using polyethyleneimine. After 48 h, medium containing the infectious virus was centrifuged, filter-sterilized, supplemented with 8 μg ml −1 polybrene and used to infect KP or H727 cells for 48 h. Cells were allowed to recover for another 48 h before adding puromycin for selection of cells stably expressing the shRNA. Puromycin-resistant cells were further sorted for high GFP (in the case of GIPZ constructs) or high red fluorescent protein (RFP) (in the case of TRIPZ constructs) expression using flow cytometry. Reporter assay Stable HeLa clones bearing an array of amplified Collagenase–Luciferase gene units were obtained by blasticidin selection after co-transfection of equimolar amounts of −517/+63 Collagenase-Luc [55] , [56] and pΔBN-AR1, which promotes an amplification of co-transfected plasmids [57] . Cells were plated in 24 wells and transfected with 250 ng shRNA constructs with 50 ng Ubiquitin-Renilla as an internal control. After 48 h the cells were lysed and luciferase activity was measured using the Dual Luciferase reporter assay (Promega), as per the manufacturer’s instructions. qRT–PCR on cell lines RNA was extracted from cells using the Qiagen RNAeasy mini kit, DNase-treated (Ambion) and cDNA-synthesised using Superscript III (Invitrogen) according to the manufacturer’s instructions. QPCR was performed using a ABIPrism 7500HT sequence detection system with SYBR Green incorporation. QPCR primers were as follows: mouse Trim7, forward: 5′-cagctcaactgtgggcact-3′, reverse: 5′-gcatgtcctccactgcatag-3′; mouse c-Jun, forward: 5′-tgaaagctgtgtcccctgtc-3′, reverse: 5′-atcacagcacatgccacttc-3′; mouse cyclin D1, forward: 5′-gtgcgtgcagaaggagattgt-3′, reverse: 5′-ctcacagacctccagcatcca-3′; mouse HB–EGF, forward: 5′-tgctgccgtcggtgatg-3′, reverse: 5′-caccaacgcggacaacact-3′; mouse cdc2, forward: 5′-ggacgagaacggcttggat-3′, reverse: 5′-attcgtttggcaggatcatagac-3′; mouse CD44, forward: 5′-ctcctggcactggctctga-3′, reverse: 5′-ctgcccacaccttctcctactatt-3′; mouse β-actin, forward: 5′-atgctccccgggctgtat-3′, reverse: 5′-cataggagtccttctgacccattc-3′, human Trim7, forward: 5′-ttctccagcttctgggtagc-3′, reverse: 5′-cgctgagcagggagtagc-3′; human c-Jun, forward: 5′-ccaaaggatagtgcgatgttt-3′, reverse: 5′-ctgtccctctccactgcaac-3′; human CyclinD1, forward: 5′-agctcctgtgctgcgaagtggaaac-3′, reverse: 5′-agtgttcaatgaaatcgtgcggggt-3′; human cdc2, forward: 5′-tggatctgaagaaatacttggattcta-3′, reverse: 5′-caatcccctgtaggatttgg-3′; human CD44, forward: 5′-tgccgctttgcaggtgat-3′, reverse: 5′-ggcctccgtccgagaga-3′; human MSK1, forward: 5′-tgctgacagattttggtctga-3′, reverse: 5′-atagttccacaaaaggaatatgctc-3′; human MSK2, forward: 5′-cacgaggtgcatcacgac-3′, reverse: 5′-gctgaagtgccgcttctt-3′; human Actin, forward: 5′-tggatcagcaagcaggagtat-3′, reverse: 5′-gcatttgcggtggacgat-3′. All primer pairs generated a single PCR product, as determined by dissociation curve analysis. Immunoprecipitations HEK293T cells expressing Myc–Trim7 with or without FLAG–RACO-1 were lysed with Buffer A (0.2% NP-40, 150 mM NaCl, 20 mM Tris pH 7.5, 500 μM EDTA, protease inhibitor cocktail (Sigma), 100 μM phenylmethyl sulphonyl fluoride (PMSF), 1 mM Na 3 VO 4 , 50 mM NaF, 1 mM β-glycerophosphate and 1 mM dithiothreitol (DTT)) and subjected to Flag immunoprecipitation with anti-Flag agarose beads (A2220, Sigma). For coimmunoprecipitation of GFP–RACO-1 with Myc–Trim7, 293T cells expressing Myc–Trim7 and WT or deletion mutant GFP–RACO-1 were lysed in buffer A and then subjected to Myc immunoprecipitation with anti-Myc agarose beads (A7470, Sigma). In vivo and in vitro ubiquitination assays For in vivo ubiquitination assays, His–Ubiquitin was affinity-purified with Ni 2+ -NTA agarose beads [58] . Briefly, FLAG–RACO-1 and His–Ubiquitin with or without Myc–Trim7 were transfected in 293T cells. Cells were lysed in buffer B (100 mM sodium phosphate pH 8.0, 5 M guanidinium hydrochloride) containing 10 mM imidazole. Ubiquitinated proteins were precipitated using Ni 2+ -NTA agarose beads (Qiagen). Beads were washed three times in buffer B containing 20 mM imidazole, and then three times in buffer containing 1 M guanidinium hydrochloride and finally three times in buffer C (25 mM Tris pH 6.5, 20 mM imidazole). Proteins were eluted from the beads by addition of 250 mM imidazole and were subjected to western blotting. For in vitro ubiquitination, FLAG–RACO-1 was immunoprecipitated from Trim7-depleted HEK293T cells using anti-FLAG M2 agarose beads (Sigma), washed with buffer A containing 1 M NaCl, and then with buffer A containing no NaCl and finally with buffer A containing 150 mM NaCl. Immunoprecipitated protein was eluted with 100 ng ml −1 3X-FLAG peptide (Sigma). Eluted FLAG–RACO-1 was incubated with 50 nM UBE1, 500 nM UbcH5a, 5 μM HA–Ubiquitin and GST–Trim7 wt or mutants in buffer E (50 mM Tris-Cl pH 8.0, 10 mM MgCl 2 , 2 mM DTT and 4 mM ATP) for 2 h at 30 °C. Reactions were stopped by addition of SDS loading dye and subjected to western blotting with RACO-1 antibody as above. Protein purification GST–Trim7 wt or mutant expression vectors were transformed into BL21 (DE3) bacteria and a single colony expanded. Cultures were grown to an optical density of 0.6 and protein expression was induced by the addition of 1 mM isopropyl-b-D-thiogalactoside for 4 h at 37 °C. Pelleted bacteria were lysed by sonication in Buffer D (20 mM Tris pH 7.5, 150 mM NaCl, 0.5% Triton X-100, 100 μM PMSF, 5 mM β-mercaptoethanol and 10% glycerol). Fusion proteins were isolated by affinity purification using Glutathione Sepharose 4B beads (Amersham), washed four times with Buffer D containing 2 mM glutathione and then the protein was eluted by 20 mM glutathione. Purified protein was dialysed against buffer D to remove glutathione before storage. The construct encoding the mouse C-terminal activation domain of Elk-1 (GST-(His) 6 -Elk-1 residues 309–429) was inserted into the BamHI–NotI cloning sites of pET-41a (ref. 59 ) and expressed in Escherichia coli strain BL21(DE3; Novagen) as an N-terminal GST-(His) 6 fusion protein. For the purification of the bacterially expressed GST-(His) 6 -Elk-1 309–429 construct, cells were lysed in buffer E (50 mM Tris pH 8.0, 300 mM NaCl and 5 mM DTT) with complete protease inhibitor cocktail (Roche Diagnostics). The cleared lysate was applied to glutathione sepharose resin (GE Healthcare Life Sciences), washed extensively first with buffer E and finally with buffer F (50 mM Tris pH 8.0, 150 mM NaCl and 5 mM DTT). The GST-(His) 6 tag was cleaved overnight by incubating the protein with 1:50 (w/w) GST-3C protease on the resin. Cleaved protein was collected and further purified on a Superdex 75 HR10/30 size exclusion column (GE Healthcare Life Sciences) in buffer G (25 mM Tris pH 7.5, 150 mM NaCl). Constitutively active ERK2 was expressed in bacteria as an N-terminal (His) 6 fusion protein and purified using the protocol described in ref. 60 . Briefly, expression of recombinant ERK2 was induced with 0.25 mM isopropyl-β- D -thiogalactopyranoside at 30 °C for 12–14 h. Cells were lysed in buffer H (50 mM sodium phosphate, pH 8.0, 0.3 M NaCl) with complete protease inhibitor cocktail (Roche Diagnostics). The lysate was clarified at 20,000 g for 30 min at 4 °C. The resulting supernatant was applied to Ni 2+ -NTA resin equilibrated in buffer H, washed with 20 volumes of buffer I (20 mM Tris-HCl, pH 8.0, 0.3 M NaCl and 10 mM imidazole) and eluted with 0.25 M imidazole, pH 7.0, in buffer I. Eluted protein was dialysed overnight against buffer J (20 mM Tris-HCl, pH 7.5, 50 mM NaCl, 1 mM DTT and 1 mM EGTA), applied to a Mono Q column (GE Healthcare) equilibrated in the same buffer and eluted with 500 mM NaCl in buffer I. Fractions containing purified ERK2 were pooled, dialysed against buffer I containing 20% glycerol and protease inhibitors, frozen in liquid nitrogen and stored at −80 °C in small aliquots. In vitro kinase assay For ERK kinase activity, GST or GST–Trim7 or Elk-1 was incubated with ERK2 in buffer K (50 mM Tris-Cl pH 8.0, 150 mM NaCl, 10 mM MgCl 2 , 1 mM EDTA and 2 mM DTT) containing 0.2 mM ATP and 20 μCi γ 32 P ATP for 1 h at 30 °C. The reaction was stopped by adding SDS loading dye and analysed on SDS–PAGE. The gel was dried and bands were visualized with autoradiography. For MSK1 kinase reaction, FLAG–MSK1 WT or FLAG–MSK1 D565A were ectopically expressed in 293T cells, immunoprecipitated by anti-FLAG M2 agarose beads (Sigma), washed and eluted using 100 μg ml −1 3 × FLAG peptide (Sigma). Eluted MSK1 or MSK1 D565A was incubated with GST–Trim7 or GST–CREB in buffer H containing 20 μM ATP and 20 μCi γ 32 P ATP for 1 h at 30 °C. The reactions were analysed as described above. Ethical considerations Experiments using mice ( Mus musculus ) were carried out with the approval of the London Research Institute’s Ethical Review Committee according to the UK Animals (Scientific Procedures) Act 1986. For the lung cancer model, animals were culled 12 weeks after intubation, before tumours outwardly affect the health of the animal. For xenograft experiments, subcutaneous tumours were allowed to reach a maximum of 1.4 cm in length before the experiment was terminated. Generation of transgenic mice The conditional ROSA26-Trim7-IRES-eGFP-pA+ targeting vector (using human cDNA sequence for Trim7 isoform 1) was generated through LR reactions between the pDONR-Trim7 and the Gateway compatible pROSA26-DV1 plasmids [61] . The ROSA26-Trim7 conditional targeting vector was linearized with Pvu1 and electroporated into the G4 ES cell line [62] , and ES clones were selected by G418 resistance and screened by PCR analysis [61] . Correctly targeted ROSA26-Trim7 ES cell clones were aggregated with WT Swiss diploid host embryos and strong male chimeras were generated that transmitted the conditional ROSA26-Trim7-IRES-eGFP-pA+ transgene to F1 generation offspring [61] . These mice were then bred with the K-Ras G12D mouse model [26] , [27] to generate KT mice. Adenoviral infection Adeno-Cre virus (Ad5CMVCre) was purchased from the Gene Transfer Vector Core, University of Iowa. Intratracheal intubation [26] was carried out on animals at 8–12 weeks of age using a dose of 2.5 × 10 7 viral particles per mouse. Briefly, the adenovirus was prepared in MEM and 10 mM calcium chloride was added and allowed to precipitate at room temperature. The mouse was anaesthetized and the virus preparation was administered via a catheter inserted into the trachea. Both male and female transgenic mice were used. A sample size of at least five mice per genotype was used to allow statistical analysis to be performed, with no sample exclusion criteria. Mice were culled 12 weeks after intubation for analysis. Immunohistochemistry and qRT–PCR on transgenic mouse tissue Mice were killed by cervical dislocation and lungs were perfused with PBS and then with 10% neutral buffered formalin (NBF). Lung tissue was incubated in 10% NBF overnight and washed with 70% ethanol. Paraffin-embedded 4-μM sections were stained with the following antibodies: TTF-1 (ab40880, Abcam), GFP (ab290, Abcam), Surfactant Protein C (AB3786, Millipore), c-Jun (610326, BD Biosciences) and Ki67 (M7248, DAKO). All the antibodies were used at 1:100 dilution for immunohistochemistry. TTF-1 was used as a marker of lung adenocarcinoma to differentiate transformed from untransformed lung tissue. The ImageJ software was used to quantify the TTF-1-positive transformed lung area. Lungs from 5 R26Trim7 , 9 K-Ras G12D and 12 KT mice were analysed. Each data point in Fig. 5e represents one mouse. For Ki67 or c-Jun staining, the entire lung section was imaged using a Nanozoomer (Hamamatsu) slide scanner. The tumour areas were outlined and Ki67- or c-Jun-positive and -negative nuclei were quantified automatically with the APPsolute Digital Pathology software (VisioPharm) using a standard threshold staining intensity. For each tumour, the number of Ki67- or c-Jun-positive cells was calculated and represented as percentage of total number of cells. Five mice of each genotype were used; in total, 36 K-Ras G12D and 243 KT tumours were analysed for Ki67 staining and 43 K-Ras G12D and 151 KT tumours were analysed for c-Jun staining. Each data point in Fig. 5g,i represents one tumour. For RNA and protein isolation, lungs were perfused with PBS and minced and then resuspended in DMEM containing collagenase type III and incubated for 30 min at 37 °C in a shaking incubator. Cells were centrifuged for 5 min at 300 g and then passed through a 70-μm cell strainer and then used for either protein preparation or RNA isolation as described above. Xenograft experiments Female NOD-SCID mice were subcutaneously injected at 8 weeks of age with shControl cells (stably transfected with shRNA construct as described above) on the left flank and shTrim7 cells on the right. A sample size of at least four mice per cohort was used to allow statistical analysis to be performed, with no sample exclusion criteria. For the ‘+Dox’ cohort, five mice received a daily dose of 5 mg ml −1 aqueous solution of doxycycline by oral gavage starting from day 25 and continuing to the end of the experiment. For the ‘no Dox’ cohort, four mice did not receive any treatment as a control. Randomization and blinding were not used. Subcutaneous tumour volumes were determined every 2 days by measuring the external dimensions of the tumour with calipers. Two perpendicular diameters were measured in each case and the longer designated ‘length’ ( L ) and the shorter ‘width’ ( W ). The tumour volume ( V ) was calculated using the following equation, taken from ref. 63 : The experiment was terminated once the largest xenograft tumour reached 1.4 cm in length, whereupon the mice were culled and the tumours excised and photographed. Mass spectrometry Biotinylated RACO-1(163–235) and scrambled peptides (2 mg) were incubated with Dynabeads M280 streptavidin in PBS at 4 °C overnight. Peptide-bound beads were washed and resuspended in buffer A. HeLa cells were lysed in buffer A and then incubated with Dynabead-bound peptides for 2 h at 4 °C. The beads were washed three times with buffer A containing 300 mM NaCl. For LC-tandem mass spectrometry (MS-MS), polyacrylamide gel slices (1–2 mm) containing the purified proteins were prepared for analysis using the Janus liquid handling system (Perkin Elmer, UK). Briefly, the excised protein gel pieces were placed in wells of a 96-well microtiter plate, destained with 50% (vol/vol) acetonitrile and 50 mM ammonium bicarbonate, reduced with 10 mM DTT and alkylated with 55 mM iodoacetamide. Alkylated proteins were digested with 6 ng μl −1 trypsin (Promega, UK) overnight at 37 °C. The resulting peptides were extracted in 1% (vol/vol) formic acid, 2% (vol/vol) acetonitrile and were analysed by nanoscale capillary LC-MS-MS using a nanoAcquity UPLC (Waters, UK) to deliver a flow of 300 nl min −1 . A C18 Symmetry 5-μm, 180-μm by 20-mm μ-precolumn (Waters) trapped the peptides before separation on a C18 BEH130 1.7-μm, 75-μm by 250-mm analytical UPLC column (Waters). The peptides were eluted with a gradient of acetonitrile. The analytical column outlet was interfaced with a Triversa NanoMate microfluidic chip for mass spectrometric analysis (Advion, UK). Mass spectrometric information was obtained using an orthogonal-acceleration quadrupole-time of flight mass spectrometer (Synapt HDMS; Waters). Data-dependent analysis was carried out, for which automatic MS-MS data on the eight most intense, multiply charged precursor ions in the m/z range of 400–1,500 were acquired. MS-MS data were acquired over the m/z range of 50–1,995. LC-MS-MS data were then searched against the UniProt KB (release 15.5) protein database using the Mascot search engine programme (Matrix Science, UK) [64] . How to cite this article: Chakraborty, A. et al. The E3 ubiquitin ligase Trim7 mediates c-Jun/AP-1 activation by Ras signalling. Nat. Commun. 6:6782 doi: 10.1038/ncomms7782 (2015).